Frequency-dependent recruitment of V2a interneurons during fictive locomotion in the mouse spinal cord The principles governing the recruitment of interneurons during acceleration in vertebrate locomotion are unknown. In the mouse, the V2a spinal interneurons are dispensable for left–right coordination at low locomotor frequencies, but their function is essential for maintaining left–right coordination at high frequencies. Here we explore the mechanisms driving this frequency-dependent role using four methods to determine how V2a interneurons are recruited at different locomotor frequencies. We show that half of the V2a interneurons receive rhythmic locomotor synaptic drive, which increases with cycle frequency, recruiting more of the neurons to fire at higher frequencies. The other V2a interneurons do not receive locomotion-related synaptic drive and are not recruited into the locomotor network at any frequency. The increased role of V2a interneurons at higher locomotor frequencies arises from increased synaptic drive to recruit subthreshold oscillating V2a neurons, and not from recruitment of a second set of silent V2a interneurons. Central pattern generators (CPGs) are defined neural networks that drive simple rhythmic movements such as respiration and locomotion [1] , [2] , [3] , [4] , [5] , [6] . Research in simpler invertebrate CPGs has shown that the neuronal composition of the network can change under different conditions, to drive variants on the basic behaviour [7] , [8] . In vertebrate locomotor CPGs, which are located in the spinal cord, recent research has addressed the question of whether the neuronal composition of the CPG changes as the speed of locomotion increases. Studies of motoneuron activity demonstrate the size principle for recruitment in many species [9] , [10] , [11] : smaller motoneurons, with higher input resistance, are recruited at lower locomotor speeds, whereas larger motoneurons, with lower input resistance, are only recruited at higher speeds. Recent studies of larval zebrafish have demonstrated the speed-dependent recruitment of spinal interneurons in the swim CPG [12] , [13] , [14] , [15] , [16] , [17] , [18] . As with motoneurons [12] , [13] , interneurons with higher input resistance are recruited during slow swimming whereas interneurons with lower input resistance are only recruited during fast swimming. However, unlike motoneuron recruitment, each interneuron operates only over a limited swim frequency. For example, more ventral alx -expressing Circumferential Descending (CiD) interneurons fire at lower frequencies but are actively inhibited at higher frequencies, whereas more dorsal CiD interneurons are silent at lower frequencies and are only activated at higher frequencies. These results suggest that the neuronal composition of the CPG changes with cycle frequency. In the mouse spinal cord, studies of genetically identified interneurons suggest that they have different roles at different locomotor speeds [19] . However, it is not known whether similar principles for interneurons recruitment hold in tetrapod locomotor CPGs as in the zebrafish. We have studied the velocity-dependent roles of the spinal V2a interneurons, which selectively express the Chx10 transcription factor [20] , [21] , [22] . The V2a interneurons are glutamatergic, ipsilaterally projecting neurons, which are rhythmically active during NMDA and serotonin (5-HT)-induced fictive locomotion in the isolated neonatal spinal cord [21] , [22] , [23] , [24] , [25] , [26] . Genetic deletion of V2a interneurons in Chx10::DTA mice has shown that the V2a interneurons are not essential for locomotor rhythm generation, but have a velocity-dependent role in left–right limb alternation [23] , [24] . Normal mice running on a treadmill never change gait, but use the same left–right alternating limb gait at all locomotor speeds. In contrast, Chx10::DTA mice show normal left–right alternation at low speeds but gradually shift to left–right synchronous bounding at high speeds [24] . This shift is also seen during fictive locomotion in the isolated Chx10::DTA spinal cord, suggesting that the V2a interneurons have a critical role in maintaining left–right limb alternation, but primarily at faster locomotor speeds. We previously showed that V2a interneurons fire more rhythmically at higher cycle frequencies during NMDA/5-HT-induced fictive locomotion [26] . However, the mechanisms underlying the velocity-dependent role of V2a interneurons in left–right coordination are not known. Here we pursue this question by analysing changes in the firing of individual V2a interneurons as the cycle frequency is changed in the preparation. We utilize both artificial NMDA/5-HT activation of fictive locomotion, and a more natural method of evoking fictive locomotion by stimulating descending reticulospinal pathways from the brainstem. We show that only half of the V2a interneurons are rhythmically active during fictive locomotion. These neurons increase their activity as the cycle frequency increases, because of enhanced synaptic drive from the CPG. The remaining V2a interneurons, which do not receive rhythmic synaptic drive at low locomotor frequencies, are not recruited at higher frequencies. Thus, the frequency-dependent role of the V2a interneurons appears to arise from a frequency-dependent increase in synaptic drive from the locomotor network. Firing patterns during BES-induced fictive locomotion Our previous study showed that the percentage of rhythmic V2a interneurons increases at higher cycle frequencies [26] . Here we ask, which V2a interneurons are recruited at higher frequency, and how? To address the velocity dependence of V2a interneuron recruitment, we developed methods to monitor the activity of single V2a interneurons during fictive locomotion at increasing frequencies. In addition, we used a more natural mechanism to evoke fictive locomotion by brainstem electrical stimulation (BES) [27] , [28] , [29] , which uses synaptic pathways rather than nonspecific bath application of neurotransmitters to activate the CPG network. Using the whole-cord/brainstem preparation, with the dorsal surface of the L2 segment removed to allow whole-cell recording of V2a interneurons, we first tested whether V2a interneurons fire rhythmically during BES-induced fictive locomotion. We monitored locomotor-like activity with extracellular recordings of the ipsilateral L 2 ventral root. Fictive locomotion was triggered during tonic BES (2–4 Hz, 4–5 ms, 1–5 mA, 1- to 1.5-s duration) from 41 out of 60 cords. The ventral root initially displayed tonic activity before rhythm onset; the delay from beginning of BES to onset of rhythmic activity varied from 3.1 to 8.2 s (4.6±2.9 s; n =41 cords). The cycle frequency ranged from 0.15 to 0.72 Hz (0.34±0.13 Hz; n =41 cords). In addition to tonic BES, we induced short locomotor bouts following a brief high-frequency BES, in 8 of 21 preparations. These bouts began with high cycle frequencies and slowed down over several cycles before the bout terminated. We recorded activity of 66 V2a interneurons during BES by removing the dorsal half of the L2 spinal segment in a P0–P2 Chx10-CFP spinal cord. A total of 89% (59/66) of V2a interneurons were depolarized during tonic BES (6.5±3.5 mV). The remaining seven V2a interneurons received barrages of large inhibitory postsynaptic synaptic currents (IPSCs) during tonic BES. V2a interneurons could be classified into four classes during tonic BES-induced fictive locomotion ( Fig. 1 ). A total of 53% (35 of 66) of V2a interneurons showed rhythmic activity at a fixed phase with the iL2 motoneuron bursts ( Fig. 1a,b ), whereas 47% (31 of 66) did not show rhythmic activity ( Fig. 1c,d ). The rhythmically active V2a interneurons could be subdivided into a rhythmically firing V2a group that fired rhythmic bursts of action potentials (80%; n =28/35), and a subthreshold rhythmic V2a group that received rhythmic synaptic drive but did not fire action potentials (20%; n =7/35). The firing phase of the rhythmically spiking neurons was analysed by circular plot analysis ( Fig. 1e ). These rhythmic interneurons did not fire tight clusters of action potentials; instead, they tended to fire broadly during one half of the locomotor cycle ( Fig. 1e ). 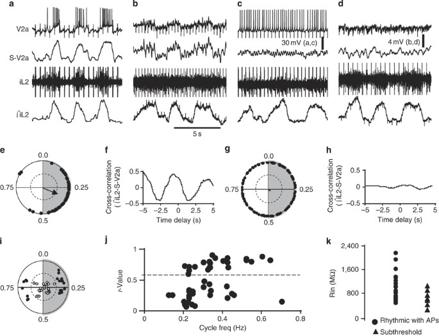Figure 1: Firing patterns of V2a interneurons during tonic BES-induced fictive locomotion. (a) Recording of a rhythmically firing V2a interneuron and its associated L2 ventral root activity during tonic BES-induced fictive locomotion. The smoothed neuronal trace (S-V2a) is shown below the real recording. The ventral root activity is integrated and smoothed and shown under the VR recordings (∫iL2). (b) Recording of a subthreshold rhythmic V2a interneuron and the associated L2 ventral root activity during tonic BES-induced fictive locomotion. (c) Recording of a non-rhythmic tonically firing and L2 ventral root activity during tonic BES-induced fictive locomotion. (d) Recording of a silent V2a interneuron and L2 ventral root activity during tonic BES-induced fictive locomotion. (e) Circular plot of activity of theV2a interneuron froma. The grey area indicates the ipsilateral L2 activity phase in the cycle. (f) Cross-correlogram of the smoothed membrane potential oscillations of the subthreshold V2a interneurons with the rectified and smoothed ventral root output fromb. (g) Circular plot of activity of the V2a interneuron fromc. The grey area indicates the ipsilateral L2 activity phase in the cycle. (h) Cross-correlogram of the smoothed membrane potential oscillations of the silent V2a interneurons and the rectified and smoothed ventral root output fromd. (i) Summary of the firing phase and rhythmicity of all V2a interneurons that fired action potentials during BES-induced fictive locomotion. The dashed line shows ther-value for statistically significant rhythmicity. Filled circles: significantly rhythmic (as ina); open circles, not rhythmic (as inc). (j) Relationship between locomotor cycle frequency and circular plotr-values of 45 V2a interneurons during tonic BES-induced fictive locomotion. The dashed line indicates ther-value for statistically significant rhythmicity. (k) Subthreshold V2a interneurons have lower input resistance than those that fire action potentials during low-frequency BES-induced fictive locomotion. The neuron in Figure 1a,e fired in phase with the ipsilateral L2 motoneuron burst, which represents the flexor phase of the motor pattern. The subthreshold rhythmicity in this group can be detected by the cross-correlation between the smoothed membrane potential oscillations and the rectified and smoothed ventral root output ( Fig. 1f ). Figure 1: Firing patterns of V2a interneurons during tonic BES-induced fictive locomotion. ( a ) Recording of a rhythmically firing V2a interneuron and its associated L2 ventral root activity during tonic BES-induced fictive locomotion. The smoothed neuronal trace (S-V2a) is shown below the real recording. The ventral root activity is integrated and smoothed and shown under the VR recordings (∫iL2). ( b ) Recording of a subthreshold rhythmic V2a interneuron and the associated L2 ventral root activity during tonic BES-induced fictive locomotion. ( c ) Recording of a non-rhythmic tonically firing and L2 ventral root activity during tonic BES-induced fictive locomotion. ( d ) Recording of a silent V2a interneuron and L2 ventral root activity during tonic BES-induced fictive locomotion. ( e ) Circular plot of activity of theV2a interneuron from a . The grey area indicates the ipsilateral L2 activity phase in the cycle. ( f ) Cross-correlogram of the smoothed membrane potential oscillations of the subthreshold V2a interneurons with the rectified and smoothed ventral root output from b . ( g ) Circular plot of activity of the V2a interneuron from c . The grey area indicates the ipsilateral L2 activity phase in the cycle. ( h ) Cross-correlogram of the smoothed membrane potential oscillations of the silent V2a interneurons and the rectified and smoothed ventral root output from d . ( i ) Summary of the firing phase and rhythmicity of all V2a interneurons that fired action potentials during BES-induced fictive locomotion. The dashed line shows the r -value for statistically significant rhythmicity. Filled circles: significantly rhythmic (as in a ); open circles, not rhythmic (as in c ). ( j ) Relationship between locomotor cycle frequency and circular plot r -values of 45 V2a interneurons during tonic BES-induced fictive locomotion. The dashed line indicates the r -value for statistically significant rhythmicity. ( k ) Subthreshold V2a interneurons have lower input resistance than those that fire action potentials during low-frequency BES-induced fictive locomotion. Full size image In contrast to the rhythmic V2a interneurons, 47% of V2a neurons did not show any rhythmic activity during BES-evoked fictive locomotion. These non-rhythmic V2a neurons could also be divided into two groups: one group fired tonic action potentials with no rhythmicity ( n =14; Fig. 1c ), as seen in the circular plot in Figure 1g , whereas the other group remained silent and showed no subthreshold rhythmic input ( n =8; Fig. 1d,h ). Figure 1i summarizes the mean phase and rhythmicity of all 46 V2a interneurons that fired action potentials during BES-induced fictive locomotion. The filled circles represent neurons that showed rhythmic firing activity, as in Figure 1a . As is seen during NMDA/5-HT-evoked fictive locomotion [25] , [26] , V2a interneurons could fire either in phase (flexor related: filled circles with phases between 0 and 0.5) or antiphase (extensor related: circles with phases between 0.5 and 1.0) with iL2 ventral root activity. We investigated whether the rhythmicity of the V2a neurons during BES-induced fictive locomotion is related to the locomotor cycle frequency. As shown in Figure 1j , there was a significant positive relationship between the cycle frequency and the r -value obtained from circular plot analysis, which reflects the degree of rhythmic clustering of the action potentials of a V2a interneuron during a specific phase of the locomotor cycle ( R =0.4; P =0.006; n =46 actively firing interneurons, non-zero correlation between cycle frequency and r -value). More V2a interneurons fire rhythmically at higher frequencies ( Fig. 1j ). When the locomotor frequency is faster than 0.4 Hz, 64% of V2a neurons (9 out 14) are rhythmic; when the locomotor frequency is <0.4 Hz, only 40% (13 out 32) are rhythmic. This positive relationship between cycle frequency and V2a rhythmicity during BES-induced fictive locomotion parallels our previous results using NMDA/5-HT to induce fictive locomotion [24] , [26] , suggesting that it is unlikely to be an artefact of transmitter bath application. As described previously [25] , [26] , V2a interneurons show variable intrinsic electrophysiological properties, firing either tonically, phasically or with a delay in response to a depolarizing current step. There was no obvious relationship between the intrinsic firing properties of V2a interneurons and their activity during BES-induced fictive locomotion: the tonic, phasic or delayed V2a interneurons could be either rhythmic or non-rhythmic. We next asked whether the recruitment of rhythmically active V2a interneurons varies with their input resistance, as predicted by the size principle [9] , [10] , [11] . The input resistance of rhythmic V2a interneurons varied from 256 to 2109 MÙ; the two rhythmically active populations had a mean input resistance of 873±425 MΩ ( n =35). In this rhythmic population, the subthreshold rhythmic V2a neurons had a significantly lower input resistance (652±267 MΩ; n =7) than the rhythmically firing V2a interneurons (938±445 MΩ; n =28; P <0.005 unpaired t -test; Fig. 1k ). Thus, input resistance may have a role in determining the recruitment pattern of V2a interneurons during fictive locomotion. These results show that during either NMDA/5-HT-induced or tonic BES-induced fictive locomotion, a higher percentage of V2a interneurons fires rhythmically at higher cycle frequencies. However, this does not show how the neurons are recruited as the cycle frequency accelerates, which requires that we monitor the activity of single V2a interneurons as the locomotor frequency changes. Below we describe four different ways to accomplish this goal. V2a recruitment with increased NMDA/5-HT concentration In our first method, fictive locomotion was first triggered by low concentrations of NMDA/5-HT; after the rhythmic motor pattern had stabilized, the concentrations of NMDA/5-HT were slightly elevated. This often increased the cycle frequency. 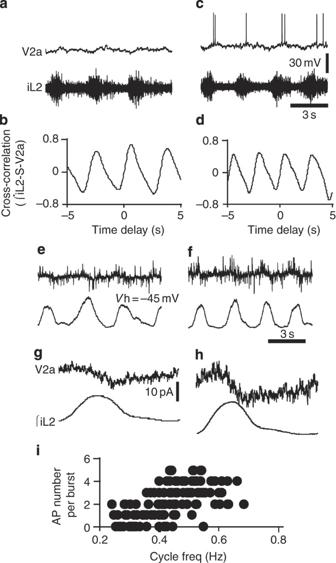Figure 2: Subthreshold V2a interneurons during low-frequency fictive locomotion are recruited at higher frequencies. (a) Activity of a subthreshold V2a interneuron and the associated ipsilateral ventrol root activity during fictive locomotion induced by 8-μM NMDA and 8-μM 5-HT. (b) The cross-correlogram between the smoothed membrane potential oscillations of the V2a interneurons and the rectified and smoothed ventral root output froma. (c) Recording of the same V2a interneuron and ventral root at a higher locomotor frequency after raising the NMDA/5-HT concentrations to 10 μM each. (d) The cross-correlogram between the smoothed membrane potential oscillations of the V2a interneurons and the rectified and smoothed ventral root output fromc. (e) Current traces of the same V2a interneuron using voltage-clamp recording at lower fictive locomotor frequencies. This is shown beneath the voltage-clamp trace. (f) Current traces of the same V2a interneuron using voltage-clamp recording at higher fictive locomotor frequencies, as shown by the smoothed and rectified ventral root activity below the trace. (g) Averaged current oscillation of the V2a interneuron at the lower cycle frequency. (h) Averaged current oscillation of the V2a interneuron during a single cycle (shown by integrated ventral root activity beneath it) at the higher cycle frequency. (i) Relationship between the action potential number per cycle and the locomotor cycle frequency for this interneuron. Figure 2a shows a V2a interneuron that exhibited subthreshold locomotor-related membrane oscillations in 8-μM NMDA/5-HT, as seen by the cross-correlation of its smoothed membrane potential with the smoothed and rectified iL2 ventral root bursts ( Fig. 2b ). When the concentrations of NMDA/5-HT were increased to 10 μM, the locomotor frequency increased by 31% ( Fig. 2c ). A negative bias current (−8 pA) was injected into the neuron to maintain its membrane potential at the original level before drug elevation. As shown by the cross-correlation in Figure 2d , this neuron still exhibited locomotor-related membrane oscillations, but now underlying the generation of rhythmic action potentials. This could reflect simply the increased nonspecific excitation of this and other neurons by the elevated NMDA/5-HT. To test this, we recorded the synaptic currents of the neuron during voltage clamp before and after NMDA/5-HT elevation ( Fig. 2e,f ). With higher concentrations of NMDA/5-HT, more tonic EPSCs and IPSCs appeared; however, the phasic locomotor-related synaptic inputs were even more enhanced. To measure the change in locomotor-related synaptic currents, we performed a moving bin averaging method to average the net synaptic current during one locomotor cycle. When the elevated NMDA/5-HT concentration increased the cycle frequency by 31%, the net rhythmic synaptic current was increased from 10.3 to 14.4 pA ( Fig. 2g,h ). We have recorded from three subthreshold V2a interneurons that the locomotor frequency was accelerated by increasing the concentration of NMDA/5-HT. The synaptic current was increased from 9.4±0.8 to 13±2.6 pA ( P <0.05; n =3 cords; paired t -test), indicating that the increasing neuronal excitability is likely caused by an increase of locomotor-related synaptic drive. We also measured the number of action potentials per cycle; there is a significant relationship between cycle frequency and action potential number per cycle ( Fig. 2i ; R =0.57; P <0.0001; n =131 cycles, non-zero correlation between cycle frequency and r -value). Figure 2: Subthreshold V2a interneurons during low-frequency fictive locomotion are recruited at higher frequencies. ( a ) Activity of a subthreshold V2a interneuron and the associated ipsilateral ventrol root activity during fictive locomotion induced by 8-μM NMDA and 8-μM 5-HT. ( b ) The cross-correlogram between the smoothed membrane potential oscillations of the V2a interneurons and the rectified and smoothed ventral root output from a . ( c ) Recording of the same V2a interneuron and ventral root at a higher locomotor frequency after raising the NMDA/5-HT concentrations to 10 μM each. ( d ) The cross-correlogram between the smoothed membrane potential oscillations of the V2a interneurons and the rectified and smoothed ventral root output from c . ( e ) Current traces of the same V2a interneuron using voltage-clamp recording at lower fictive locomotor frequencies. This is shown beneath the voltage-clamp trace. ( f ) Current traces of the same V2a interneuron using voltage-clamp recording at higher fictive locomotor frequencies, as shown by the smoothed and rectified ventral root activity below the trace. ( g ) Averaged current oscillation of the V2a interneuron at the lower cycle frequency. ( h ) Averaged current oscillation of the V2a interneuron during a single cycle (shown by integrated ventral root activity beneath it) at the higher cycle frequency. ( i ) Relationship between the action potential number per cycle and the locomotor cycle frequency for this interneuron. Full size image Next, we tested whether the neurons that were already firing rhythmic bursts of action potentials at low NMDA/5-HT concentrations remained silent at higher frequencies with elevated NMDA/5-HT, as previously seen with zebrafish CiD neurons [13] . 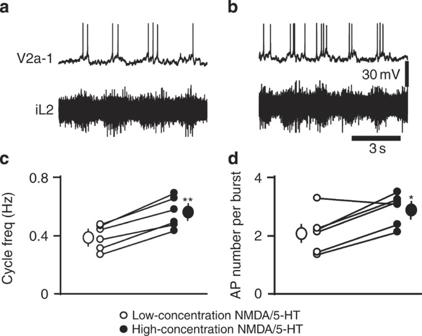Figure 3: Enhanced activity of rhythmically firing V2a interneurons with increased locomotor frequency. (a) Recording of a rhythmically firing V2a interneuron during fictive locomotion induced by 8-μM NMDA/5-HT, with ipsilateral ventral root trace shown beneath it. (b) This V2a interneuron increases its spike frequency when the NMDA/5-HT concentrations are raised to 10 μM. (c) In six cords, the locomotor cycle frequency increased as the concentration of NMDA/5-HT was increased (n=6; **P=0.0013, pairedt-test). Larger circles show mean values at lower and higher drug concentrations. (d) V2a action potential number per cycle is increased in five of six neurons after increasing the NMDA/5-HT concentration (n=6; *P=0.007). Data are expressed as mean±s.d. Figure 3a shows one V2a interneuron that was rhythmically active at relatively low frequencies during NMDA/5-HT-induced fictive locomotion. When the frequency was increased with elevated NMDA/5-HT, this V2a interneuron continued to fire action potentials with an increased number of spikes per cycle ( Fig. 3b ). We measured six V2a interneurons that showed rhythmic firing during fictive locomotion induced by different concentrations of NMDA/5-HT. The average locomotor cycle frequency increased from 0.38±0.1 to 0.54±0.1 Hz ( Fig. 3c ; P <0.001; n =6; paired t -test), whereas the action potential number per cycle was significantly enhanced in five of the six neurons, with a mean increase from 2.1±0.7 to 2.9±0.6 ( Fig. 3d ; P <0.01; n =6; paired t -test). Figure 3: Enhanced activity of rhythmically firing V2a interneurons with increased locomotor frequency. ( a ) Recording of a rhythmically firing V2a interneuron during fictive locomotion induced by 8-μM NMDA/5-HT, with ipsilateral ventral root trace shown beneath it. ( b ) This V2a interneuron increases its spike frequency when the NMDA/5-HT concentrations are raised to 10 μM. ( c ) In six cords, the locomotor cycle frequency increased as the concentration of NMDA/5-HT was increased ( n =6; ** P =0.0013, paired t -test). Larger circles show mean values at lower and higher drug concentrations. ( d ) V2a action potential number per cycle is increased in five of six neurons after increasing the NMDA/5-HT concentration ( n =6; * P= 0.007). Data are expressed as mean±s.d. Full size image We used a second method to increase the locomotor cycle frequency while recording from a V2a interneuron, by slowly washing in a higher initial concentration of NMDA/5-HT. In 4 of 16 cords perfused directly with 10 μM each of NMDA/5-HT, the fictive locomotor pattern was initiated at a low frequency, and gradually increased in frequency as the higher concentration stabilized ( Fig. 4a ). In these experiments, no bias currents were used. 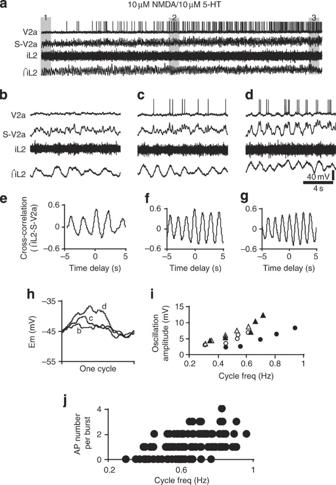Figure 4: Response of a subthreshold V2a interneuron as the locomotor cycle frequency increases during slow wash-in of 10-μM NMDA/5-HT. (a) Initiation and acceleration of bursting in a V2a interneuron as fictive locomotion accelerates during 10-μM NMDA/5-HT application. In this preparation, the fictive locomotion starts slowly and gradually increases with time. S-V2a, smoothed and filtered V2a activity; iL2, activity of the ipsilateral ventral root; ∫iL2, integrated and rectified iL2 activity. (b) Activity of this V2a interneuron at the locomotor frequency indicated by the grey area 1 ina. (c) Activity of this V2a interneuron at the locomotor frequency indicated by the grey area 2 ina. (d) Activity of this V2a interneuron at the locomotor frequency indicated by the grey area 3 ina. (e) Cross-correlogram between the smoothed V2a membrane potential oscillations and the rectified and smoothed ventral root output fromb. (f) Cross-correlograms between the smoothed V2a membrane potential oscillations and the rectified and smoothed ventral root output fromc. (g) Cross-correlograms between the smoothed V2a membrane potential oscillations and the rectified and smoothed ventral root output fromd. (h) Averaged membrane potential oscillations during one locomotor cycle fromb–d. (i) Summary of the relationship between the V2a membrane oscillation amplitude and cycle frequencies from four different cords. (j) Relationship between the action potential number per cycle of the V2 interneuron froma, and locomotor cycle frequency. As shown in Figure 4b , an initially silent V2a interneuron received rhythmic subthreshold locomotor-related synaptic drive at 0.45 Hz ( Fig. 4b ). When the cycle frequency increased to 0.6 Hz, this V2a interneuron increased its oscillations and started to fire action potentials ( Fig. 4c ). When the preparation stabilized the cycle frequency was 0.94 Hz, and the neuron increased its spike frequency further ( Fig. 4d ). In the three situations, the neuronal membrane potentials were positively correlated to the smoothed ipsilateral ventral root activity ( Fig. 4e,f,g ). Using the moving bin method, we averaged the amplitude of the V2a membrane potential oscillations at different frequencies. The oscillation amplitude gradually increased from 2.4 to 8.2 mV as the cycle frequency increased from 0.46 to 0.94 Hz ( Fig. 4h ). Similar results were obtained with other three subthreshold V2a interneurons. Averaged over these neurons, there was a significant relationship between the cycle frequency and the membrane oscillation amplitude ( Fig. 4i ; R =0.61; P =0.042; n =20 from four cords, non-zero correlation between cycle frequency and r -value). In addition, all these subthreshold V2a interneurons reached threshold and increased their spike frequency as the cycle frequency increased; there was a significant relationship between the cycle frequencies and number of action potentials per cycle ( Fig. 4j ; R =0.41; P <0.001; n =157 cycles, non-zero correlation between cycle frequency and r -value). Figure 4: Response of a subthreshold V2a interneuron as the locomotor cycle frequency increases during slow wash-in of 10-μM NMDA/5-HT. ( a ) Initiation and acceleration of bursting in a V2a interneuron as fictive locomotion accelerates during 10-μM NMDA/5-HT application. In this preparation, the fictive locomotion starts slowly and gradually increases with time. S-V2a, smoothed and filtered V2a activity; iL2, activity of the ipsilateral ventral root; ∫iL2, integrated and rectified iL2 activity. ( b ) Activity of this V2a interneuron at the locomotor frequency indicated by the grey area 1 in a . ( c ) Activity of this V2a interneuron at the locomotor frequency indicated by the grey area 2 in a . ( d ) Activity of this V2a interneuron at the locomotor frequency indicated by the grey area 3 in a . ( e ) Cross-correlogram between the smoothed V2a membrane potential oscillations and the rectified and smoothed ventral root output from b . ( f ) Cross-correlograms between the smoothed V2a membrane potential oscillations and the rectified and smoothed ventral root output from c . ( g ) Cross-correlograms between the smoothed V2a membrane potential oscillations and the rectified and smoothed ventral root output from d . ( h ) Averaged membrane potential oscillations during one locomotor cycle from b – d . ( i ) Summary of the relationship between the V2a membrane oscillation amplitude and cycle frequencies from four different cords. ( j ) Relationship between the action potential number per cycle of the V2 interneuron from a , and locomotor cycle frequency. Full size image V2a activity following brief high-frequency BES A third method to evoke varying locomotor frequencies while recording from a single V2a interneuron used brief, high-frequency BES. In 8 out of 21 cords, after a brief high-frequency BES (1–1.5 s, 10–15 Hz, 4 ms, 1–5 mA), a transient bout of fictive locomotion appeared, ranging from 9 to 16 s in duration ( Fig. 5 ). These bouts displayed a high initial cycle frequency (up to 1 Hz) immediately after cessation of BES, which then gradually slowed until the rhythm ceased ( Fig. 5a,b ). 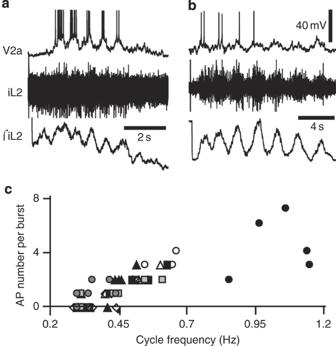Figure 5: V2a interneurons fire action potentials at the initial higher frequencies during brief BES-induced locomotor bouts. (a) Response of a rhythmic V2a interneuron during brief high-frequency BES-induced locomotor bouts. BES stimulation (10 Hz, 4 ms, 1.5 mA, 1 s duration) was applied before the start of the recording. Below the V2a recording are the iL2 and integrated iL2 recordings. The initial cycle frequency is as high as 1 Hz, and gradually decreases until the bout ceases. The interneuron is more active at the higher initial cycle frequencies. (b) Response of another rhythmic V2a interneuron during brief high-frequency BES-induced locomotor bouts. BES stimulation was applied before the start of the recording. The initial higher cycle frequency is around 0.5 Hz and gradually decreases until the bout ceases. This interneuron is also more active at the higher initial cycle frequencies. (c) Summary of relationship between action potential number per cycle and cycle frequency from eight preparations. Each shape indicates a different V2a interneuron. Eight V2a interneurons began firing rhythmic bursts of action potentials at the beginning of the transient locomotor episode; two examples are seen in Figure 5a,b . As the frequency of the transient locomotor bouts declined, these neurons fired fewer action potentials and eventually stopped firing at lower cycle frequencies. As shown in Figure 5c , there is a significant positive relationship between instantaneous cycle frequency and number of action potentials per cycle ( R =0.84; P <0.0001; n =61 cycles from eight cords, non-zero correlation between cycle frequency and r -value). Figure 5: V2a interneurons fire action potentials at the initial higher frequencies during brief BES-induced locomotor bouts. ( a ) Response of a rhythmic V2a interneuron during brief high-frequency BES-induced locomotor bouts. BES stimulation (10 Hz, 4 ms, 1.5 mA, 1 s duration) was applied before the start of the recording. Below the V2a recording are the iL2 and integrated iL2 recordings. The initial cycle frequency is as high as 1 Hz, and gradually decreases until the bout ceases. The interneuron is more active at the higher initial cycle frequencies. ( b ) Response of another rhythmic V2a interneuron during brief high-frequency BES-induced locomotor bouts. BES stimulation was applied before the start of the recording. The initial higher cycle frequency is around 0.5 Hz and gradually decreases until the bout ceases. This interneuron is also more active at the higher initial cycle frequencies. ( c ) Summary of relationship between action potential number per cycle and cycle frequency from eight preparations. Each shape indicates a different V2a interneuron. Full size image V2a activity during spontaneous locomotor frequency increases The frequency of tonic BES-induced locomotion is usually relatively constant (data not shown). However, in 3 of 28 cords, there was a spontaneous, temporary increase in cycle frequency, presumably caused by intrinsic changes in the excitability of the locomotor network ( Fig. 6a ). During these perturbations, there was a clear increase in V2a action potentials per cycle during the period of increased cycle frequencies ( Fig. 6b ). 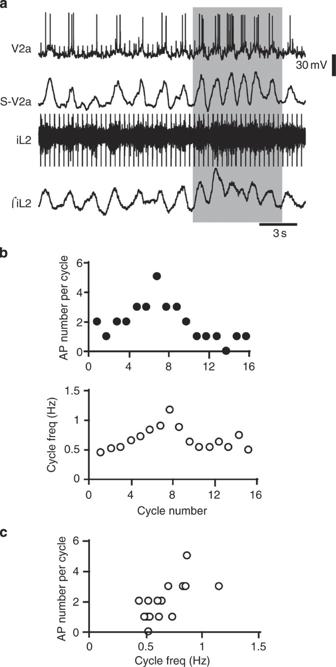Figure 6: V2a interneurons increase their firing frequency with spontaneous frequency increases during tonic BES-induced fictive locomotion. (a) Recording of a rhythmic V2a interneuron during tonic BES-induced fictive locomotion when the frequency spontaneously increased as seen in the shaded area. S-V2a, smoothed and filtered V2a activity; iL2, activity of the ipsilateral ventral root; ∫iL2, integrated and rectified iL2 activity. (b) Change in V2a action potential number per cycle and cycle frequency during each cycle of the spontaneous increase, froma. (c) Increase in action potential number per cycle as frequency spontaneously increased. During the perturbation, there is a significant relationship between the cycle frequency and the action potentials per cycle ( R =0.67; P <0.001; n =16 cycles; Figure 6c , non-zero correlation between cycle frequency and r -value). We observed a significant increase in the action potential number per cycle in two other rhythmic V2a interneurons when the frequency spontaneously increased during tonic BES-induced fictive locomotion. In the remaining rhythmic firing V2a interneurons, the locomotor cycle frequency during tonic BES was relatively stable, and no spontaneous frequency changes were observed. Figure 6: V2a interneurons increase their firing frequency with spontaneous frequency increases during tonic BES-induced fictive locomotion. ( a ) Recording of a rhythmic V2a interneuron during tonic BES-induced fictive locomotion when the frequency spontaneously increased as seen in the shaded area. S-V2a, smoothed and filtered V2a activity; iL2, activity of the ipsilateral ventral root; ∫iL2, integrated and rectified iL2 activity. ( b ) Change in V2a action potential number per cycle and cycle frequency during each cycle of the spontaneous increase, from a . ( c ) Increase in action potential number per cycle as frequency spontaneously increased. Full size image Non-rhythmic V2a neurons are not recruited at higher speeds About half of the V2a interneurons showed no rhythmic activity or synaptic drive during fictive locomotion ( Fig. 1 ). We tested whether these non-rhythmic V2a interneurons could become recruited into the locomotor pattern at higher cycle frequencies. 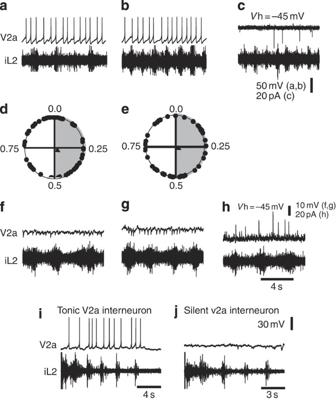Figure 7: V2a interneurons that do not receive locomotor-related synaptic drive at lower locomotor frequencies are not recruited at higher frequencies. (a) Activity of a tonically firing V2a interneuron during 8-μM NMDA/5-HT-induced fictive locomotion. (b) Increase in tonic activity but not rhythmicity after the cycle frequency is accelerated by 10-μM NMDA/5-HT. (c) Voltage-clamp recording of this V2a interneuron during fictive locomotion induced by 10-μM NMDA/5-HT. (d) Circular plot of the V2a interneuron froma, showing no rhythmicity in firing. (e) Circular plot of the V2a interneuron fromb, showing no rhythmicity in firing at the elevated cycle frequency. (f) Recording from a silent V2a interneuron during fictive locomotion induced by lower concentrations of NMDA and 5-HT (7 μM). (g) Recording from the same V2a interneuron during faster fictive locomotion induced by higher concentrations of NMDA and 5-HT (9 μM). (h) Voltage-clamp recording from this neuron during fictive locomotion induced by 9-μM NMDA/5-HT. (i) Response of a tonic V2a interneuron during a brief high-frequency BES-induced locomotor bout. (j) Response of a silent V2a interneuron during a brief high-frequency BES-induced locomotor bout. Neither neuron becomes rhythmically active. Figure 7a shows a V2a interneuron firing tonically during 8-μM NMDA/5-HT-induced fictive locomotion. When the NMDA/5-HT concentrations were increased to 10 μM each, the cycle frequency increased from 0.41 to 0.68 Hz ( Fig. 7a,b ). It did not receive any locomotor-related synaptic input measured by voltage clamp ( Fig. 7c ). This V2a interneuron fired at a higher frequency but remained tonically active at the higher cycle frequency ( Fig. 7d,e ). We characterized eight V2a interneurons that fired tonically during NMDA/5-HT-induced fictive locomotion with different frequencies; none of them became rhythmic at higher cycle frequencies. Figure 7: V2a interneurons that do not receive locomotor-related synaptic drive at lower locomotor frequencies are not recruited at higher frequencies. ( a ) Activity of a tonically firing V2a interneuron during 8-μM NMDA/5-HT-induced fictive locomotion. ( b ) Increase in tonic activity but not rhythmicity after the cycle frequency is accelerated by 10-μM NMDA/5-HT. ( c ) Voltage-clamp recording of this V2a interneuron during fictive locomotion induced by 10-μM NMDA/5-HT. ( d ) Circular plot of the V2a interneuron from a , showing no rhythmicity in firing. ( e ) Circular plot of the V2a interneuron from b , showing no rhythmicity in firing at the elevated cycle frequency. ( f ) Recording from a silent V2a interneuron during fictive locomotion induced by lower concentrations of NMDA and 5-HT (7 μM). ( g ) Recording from the same V2a interneuron during faster fictive locomotion induced by higher concentrations of NMDA and 5-HT (9 μM). ( h ) Voltage-clamp recording from this neuron during fictive locomotion induced by 9-μM NMDA/5-HT. ( i ) Response of a tonic V2a interneuron during a brief high-frequency BES-induced locomotor bout. ( j ) Response of a silent V2a interneuron during a brief high-frequency BES-induced locomotor bout. Neither neuron becomes rhythmically active. Full size image We next investigated whether silent V2a neurons, which receive only non-rhythmic inhibitory or excitatory synaptic inputs at lower locomotor cycle frequencies, could become rhythmically active at higher frequencies. Figure 7f shows a silent V2a interneuron receiving non-rhythmic inhibitory synaptic input during 7-μM NMDA/5-HT-induced fictive locomotion. This neuron remained silent when the cycle frequency was increased from 0.32 to 0.42 Hz by elevating the NMDA/5-HT concentrations from 7 to 9 μM ( Fig. 7g ). Using voltage-clamp recording, this neuron received many random IPSCs but no rhythmic synaptic inputs ( Fig. 7h ). We have monitored six V2a interneurons that were silent at lower frequencies of NMDA/5-HT-evoked fictive locomotion; none of these neurons received new rhythmic synaptic drive when the cycle frequency was elevated. We also asked whether these non-rhythmic V2a interneurons could become rhythmically active following brief high-frequency BES-induced fictive locomotor bouts. As illustrated in Figure 7i,j , neither tonically firing ( n =8 from six cords) nor silent V2a ( n =6 from four cords) interneurons showed any rhythmic activity during the BES-evoked bout of fictive locomotion. We conclude that a subset of V2a interneurons is not related to locomotion in the neonatal mouse spinal cord, and is not recruited into the motor network at any cycle frequency. During increases in locomotor speed, motoneurons follow the well-known size principle for recruitment with increasing locomotor speed or strength, but the principles for recruitment of CPG interneurons are not clear. In the zebrafish, recruitment of spinal interneurons at higher speeds is accompanied by weakening or silencing of other interneurons that were active at lower speeds [12] , [13] . Is this a generic recruitment principle for spinal interneurons? It is much more difficult to study spinal interneuron recruitment in the neonatal mouse spinal cord because of the significant difficulty in reliably altering the locomotor cycle frequency in vitro . In this study, we have used four different methods to record from V2a interneurons over a wider range of frequencies during fictive locomotion induced with either NMDA/5-HT or more naturally with BES. Our results show that only half of the V2a interneurons fire rhythmically during fictive locomotion. These neurons receive rhythmic synaptic drive, which increases with increasing cycle frequency, resulting in gradually increased recruitment and firing frequency as the locomotor cycle frequency increases. The second group of V2a interneurons does not receive rhythmic locomotor-related synaptic drive, and is not recruited into the network at any cycle frequency; they do not appear to participate in the locomotor network. The Chx10-expressingV2a interneurons recorded in this study are the homologues of the zebrafish CiD interneurons that express the Chx10 analogue alx. There are similarities and differences between the locomotor firing properties of these neurons. First, laser ablation of the more dorsally located zebrafish CiD neurons selectively disrupts high-speed swimming, altering the kinematics of the initial turn during escape turns [12] , [30] . Similarly, genetic deletion of mouse V2a interneurons selectively affects high-speed locomotion, converting the normal left–right limb alternation seen at low speeds to left–right synchrony at high speeds [24] . Second, virtually all of the spinal CiD neurons are activated during swimming episodes in the zebrafish [12] , [13] , [14] , [16] . In contrast, only half of the mouse V2a interneurons have locomotor-related activity [25] , [26] . This suggests a differentiation of subsets of V2a interneurons in tetrapods, which does not occur in the zebrafish. The function of the tonically active V2a interneurons is unknown. One possibility is that their tonic activity could contribute excitatory drive to the CPG network to support the locomotor pattern. Further experiments will be needed to determine the roles of these neurons during locomotion. Third, both the zebrafish CiD neurons and the mouse V2a interneurons are recruited roughly according to the size principle, with lower input resistance neurons firing at lower frequencies than higher input resistance neurons. However, in the larval zebrafish, CiD neurons are active only over a preferred range of locomotor frequencies, dependent on their dorsoventral location: more ventral CiDs are active at lower frequencies but actively inhibited at higher frequencies, whereas more dorsal CiDs are only active at higher frequencies. In the mouse spinal cord, the rhythmically activeV2a interneurons appear to be recruited more similar to motoneurons: virtually all increase their activity monotonically with cycle frequency. We have not observed any significant relationship between the neuronal location and V2a firing properties during fictive locomotion; Kwan et al . (2010) used calcium-imaging techniques to monitor V2a activity during fictive locomotion, and did not find any spatial clustering of rhythmically active versus tonic V2a interneurons [31] . Some V2a neurons start firing at lower frequencies and increase their activity (action potentials per cycle) as the locomotor speed accelerates ( Figs 3 and 6 ). Others are silent but receive subthreshold excitation at low frequencies and are recruited as the locomotor cycle accelerates, and then increase their firing with cycle frequency. We very rarely observed V2a interneurons that fire at higher frequencies at low cycle frequencies than at higher frequencies. An important caveat to this result, however, is that we were only able to manipulate the cycle frequency in the isolated neonatal mouse spinal cord over a limited and slow range. Mice cannot walk at birth; they do air-step or show swimming movements, but only slowly, at maximal frequencies around 1 Hz [32] . Our manipulations of fictive locomotion were within the range of 0.2–1 Hz, and thus are similar to the behavioural locomotor frequencies seen at this age. Because of technical considerations, it is not possible to study fictive locomotion in the isolated spinal cord at older ages, when the animals begin to walk normally at higher frequencies (around P14–16). Thus, it is possible that these neurons could have different frequency responses at the higher frequencies typical of adult locomotion. However, the consequences of genetic ablation of V2a interneurons were similar for adult treadmill locomotion and neonatal fictive locomotion [24] , suggesting that the frequency-dependent role of V2a interneurons in maintaining left–right alternation is preserved during postnatal maturation. In Chx10::DTA mice, which lack V2a interneurons, the speed-dependent change from left–right alternation to left–right synchrony during treadmill locomotion is not sudden. Rather, as the treadmill speed is gradually accelerated, there is a gradual transition between alternation and synchrony [24] . Similar results are obtained during fictive locomotion with the isolated Chx10::DTA spinal cord, in which the left–right phasing grades smoothly from alternation to synchrony as the cycle frequency accelerates [24] . In this study of normal V2a interneurons, we found that the rhythmic V2a interneurons increase their firing intensity by enhanced locomotor-related synaptic drive in a graded, continuous way, in agreement with the results from our genetic ablation study on neonatal and adult mice [23] , [24] . As the frequency increases, the fraction of active V2a neurons increases, the number of action potentials per cycle increases, and the clustering of the action potentials (as seen by the r -value in the circular plots) increases, all in a graded way. This gradual recruitment of V2a interneurons underlies the maintenance of left–right alternation in normal mice during acceleration from low speeds, in which V2a interneurons do not have a major role, to higher speeds, in which maintenance of left–right alternation depends on the increasing recruitment of rhythmic V2a interneurons. It may appear odd that mice have evolved this function for the V2a interneurons to prevent synchronous left–right bounding gaits, which are common in other tetrapods. It is possible that in their normal habitat, mice rarely run in a straight line for long; therefore, the benefits of bounding may be limited, and the costs of bounding in restricting the ability to suddenly change direction may have led to this function for V2a interneurons. Most previous studies of the roles of genetically identified spinal interneurons in the locomotor CPG analysed locomotion at a single speed [33] , [34] , [35] , [36] , [37] , [38] , [39] , [43] , [44] , [45] , [46] , [47] . Our work with V2a interneurons suggests that the roles of these and other interneurons may vary, depending on the locomotor speed. For example, transient inactivation of V1 interneurons reduces the locomotor speed without changing the basic pattern [19] ; these neurons may not be essential for generating the pattern, but for retaining it at high speeds. It is clear that a number of interneuron types must participate with the V2a interneurons in regulating left–right phasing; changes in their activity as the animal accelerates will complement our studies of how left–right alternation is maintained at all speeds in mice. To fully understand the specific roles of spinal interneurons in the locomotor CPG, it will be necessary to investigate their firing patterns over a wide range of locomotor speeds, although this remains a major technical challenge in the isolated mouse spinal cord. Whole-cord preparations Experiments were performed using the isolated spinal cord, with or without brainstem attached, from neonatal (postnatal (P) day P0–P4) Chx10::CFP mice. The animal protocol was approved by the Institutional Animal Care and Use Committee at Cornell University and was in accordance with National Institutes of Health guidelines. The spinal cord dissection was performed as described previously [26] . Briefly, neonatal mice were decapitated and eviscerated in cold oxygenated (95% O 2 and 5% CO 2 ) low-calcium Ringer solution composed of 111-mM NaCl, 3.08-mM KCl, 25-mM NaHCO 3 , 1.18-mM KH 2 PO 4 , 3.5-mM MgSO 4 , 0.25-mM CaCl 2 and 11-mM glucose. The spinal cord, extending from T8/T9 to S3/4, was removed and pinned dorsal-side-up in a recording chamber superfused with oxygenated Ringer solution, composed of 111-mM NaCl, 3.08-mM KCl, 25-mM NaHCO 3 , 1.18-mM KH 2 PO 4 , 1.25-mM MgSO 4 , 2.52-mM CaCl 2 and 11-mM glucose. To visualize the V2a interneurons in the spinal cord, we removed the dorsal half of the L2 segment with fine scissors during the dissection. In the brainstem–spinal cord preparation, after evisceration, a rostral cut was made between the mesencephalon and the diencephalon, and then the brainstem and spinal cord were carefully isolated, bilaterally intact. The preparation was pinned dorsal-side-up in the lumbar spinal cord region, and the brainstem was positioned ventral-side-up by twisting the thoracic/cervical segments through 180°. With these manipulations, we could record from V2a interneurons from the cut dorsal surface in the lumbar region while electrically stimulating the ventral brainstem area to trigger fictive locomotion. All experiments were performed at room temperature (20–23 °C). Electrophysiological recording V2a interneurons are located near the mid-dorsal/ventral region in lamina VII, which was visualized in the intact spinal cord preparation by removing the dorsal half of the L2 segment, as described above. In some experiments, to minimize the cut damage, only one side of the L2 dorsal segment was removed. This procedure allowed us to visualize and record from the L2 V2a interneurons during NMDA (6–10 μM)/5-HT (6–10 μM) application or during BES-induced fictive locomotion [26] . Whole-cell recordings were made with electrodes pulled from thick-walled borosilicate glass (WPI) on a vertical puller (Narishige) with resistances of 6–10 MΩ, which were lowered through the cut dorsal surface of the L2 segment. The pipette solution contained 138-mM K-gluconate, 10-mM HEPES, 5-mM ATP-Mg, 0.3-mM GTP-Li and 0.0001-mM CaCl 2 (pH was adjusted to 7.4 with KOH). The seal resistance obtained before recordings was always greater than 2 GΩ. Patch clamp recordings were made with a Multiclamp 700B amplifier (Axon Instruments) and were driven by Clampex (pClamp 9, Axon Instruments). Data were filtered at 20 kHz. BES-induced fictive locomotion Fictive locomotor activity was evoked by electrical stimulation of the brainstem. An ACSF-filled glass electrode, with a tip diameter of ∼ 100 μm, was placed on the ventral surface of the brainstem. A recording suction electrode was placed on the ipsilateral L2 (iL2) ventral root to monitor BES-induced fictive locomotion. Rhythmic burst activity from the ventral root was bandpass-filtered (100 Hz to 1 kHz). We have used two ways to trigger fictive locomotion by BES. First, tonic BES was applied (2–4 Hz, 4–5 ms, 1–5 mA). There was a short latency (typically 3–8 s) before fictive locomotion commenced. After fictive locomotion was triggered by tonic BES, the locomotor frequency did not change in a significant way when the stimulation parameters, such as frequency, duration and intensity, were varied. This is different from previous studies in rats [27] , [28] , and there could be two explanations. First, we removed the dorsal surface of the L2 segment; this manipulation may damage either the propriospinal or reticulospinal pathway, both of which are important for the BES-induced fictive locomotion. Second, the upper thoracic and cervical spinal segments were not tightly pinned down, but had to be twisted by 180° to allow simultaneous stimulation of the ventral surface of the brainstem and recording from V2a interneurons from the dorsal surface of the cord. This could damage axons descending from the brainstem to the lumbar spinal cord. The second method to induced fictive locomotion was brief high-frequency BES (10–15 Hz, 4 ms, 1–5 mA, 1–1.5 s) to induce short locomotor bouts after cessation of BES stimulation [40] . These bouts started with higher cycle frequencies and gradually slowed until the end of the bout. Correlation analysis The ventral root extracellular data were integrated and smoothed with a time constant of 0.2 s and analysed using custom-written programs in Spike 2 (Cambridge Electronic Design). The relationship between ventral root activity and neuronal membrane potential was quantified by cross-correlation analysis. Recordings were subdivided into time segments of 10 s each for the correlation analyses. Cross-correlations were computed for at least five time segments. The mean and s.e. values were obtained from the entire set. The relationship between ventral root activity and membrane potential was considered significantly rhythmic if the peak next to the centre of the average autocorrelation exceeded four times the SE of the entire set. Circular analysis Locomotor-like activity was recorded from the intact spinal cord preparation. Clampfit 9.0, Excel and Spike 2 were used for data analysis. A cycle of motor nerve activity started with the onset of an iL2 ventral root burst and ended at the onset of the next iL2 burst; these onsets were determined by a custom-made programme in Spike2 to detect when the rectified signal exceeded the average noise level between bursts by a preset amount. Data were analysed only in preparations that showed stable rhythmic ventral root activity in iL2 and in which the action potential overshoot of the Chx10 neuron was >0 mV. Individual V2a interneurons were usually recorded for >20 min during NMDA/5-HT-induced locomotor-like activity and recorded for >5 min during tonic BES-induced fictive locomotion. To determine the preferred firing phases of V2a interneurons, the phase of each spike during >35 cycles was normalized by the onset of the iL2 burst. A double-normalization process was used [41] . Circular statistics were used to determine the significance of the phasing of V2a interneurons firing during fictive locomotion [32] . The latency to each spike was measured relative to the beginning of the iL2 ventral root burst. The phase of individual spikes was determined by the latency divided by the cycle length. In each V2a interneuron, the phase of ∼ 30 spikes was measured to plot the mean vector. The direction of the mean vector represents the average preferred phase of firing of the neuron, whereas its length, r , is a measure of statistical significance of the peak preferred phase and the clustering of the spikes around the mean phase. Vectors with a phase in the range of 0.0–0.5 corresponded to cells firing in phase with iL2. P -values for the significance of r were calculated as previously described [42] . V2a interneurons were defined as rhythmic if P <0.05, by the Rayleigh test. To identify the change of synaptic currents or membrane potential, a moving average of the membrane activity traces was performed at different concentrations of NMDA/5-HT. The locomotor cycle start and end times were normalized to 0 and 1, respectively; to reduce the nonspecific synaptic events, we averaged the data from 15 locomotor cycles to test whether the locomotor-related synaptic events change at different frequencies. How to cite this article: Zhong, G. et al . Frequency-dependent recruitment of V2a interneurons during fictive locomotion in the mouse spinal cord. Nat. Commun. 2:274 doi: 10.1038/ncomms1276 (2011).